Mouse oocytes depend on BubR1 for proper chromosome segregation but not for prophase I arrest Mammalian female meiosis is error prone, with rates of meiotic chromosome missegregations strongly increasing towards the end of the reproductive lifespan. A strong reduction of BubR1 has been observed in oocytes of women approaching menopause and in ovaries of aged mice, which led to the hypothesis that a gradual decline of BubR1 contributes to age-related aneuploidization. Here we employ a conditional knockout approach in mouse oocytes to dissect the meiotic roles of BubR1. We show that BubR1 is required for diverse meiotic functions, including persistent spindle assembly checkpoint activity, timing of meiosis I and the establishment of robust kinetochore–microtubule attachments in a meiosis-specific manner, but not prophase I arrest. These data reveal that BubR1 plays a multifaceted role in chromosome segregation during the first meiotic division and suggest that age-related decline of BubR1 is a key determinant of the formation of aneuploid oocytes as women approach menopause. Missegregations during the meiotic divisions lead to the generation of aneuploid gametes that can ultimately give rise to aneuploid embryos. In humans, most aneuploidies of autosomes are lethal and result in spontaneous abortions during the first trimester. One example of a viable aneuploidy is trisomy 21, which in most cases is due to the missegregation of chromosome 21 in female meiosis I (ref. 1 ). Why female meiosis is particularly error prone, and why the rate of missegregations rises sharply with the age of the mother remains poorly understood. One reason put forward is the fact that human oocytes remain arrested for decades in prophase I before entering the meiotic divisions [2] . In addition it has been shown in mice that the cohesin complex holding sister chromatids together, is hardly renewed during oocyte growth and deteriorates with time, leading to precocious sister chromatid separation and destablization of chiasmata [3] , [4] , [5] , [6] , [7] . As in somatic cells, the spindle assembly checkpoint or SAC verifies whether all the kinetochores are correctly attached to the bipolar spindle, in mouse oocytes [8] , [9] , [10] , [11] , [12] , even though SAC control seems to be less stringent in oocytes than in somatic cells and does not seem to recognize a single unattached kinetochore [13] . In mitosis it has been shown that in the case of an unattached kinetochore, the SAC prevents metaphase-to-anaphase transition through the recruitment of SAC proteins to this kinetochore. This leads to the formation of the mitotic checkpoint complex (MCC), consisting of Cdc20, BubR1, Bub3 and Mad2, which inhibits the activation of the anaphase promoting complex/cyclosome (APC/C) and therefore the degradation of securin and cyclin B, the activation of separase and anaphase onset [14] . In meiosis, Bub1, Mps1 and Mad2 have all been shown to be essential for SAC-induced metaphase I arrest by preventing the activation of the APC/C [8] , [9] , [10] , [11] , [12] . Furthermore, SAC proteins are required for the correct timing of the extremely long prometaphase I, and meiosis I is accelerated in oocytes without functional Bub1 (ref. 8 ) or Mps1 (ref. 12 ) or when heterozygote for MAD2 (ref. 10 ). BubR1 is essential for the mitotic SAC [15] and recognizes kinetochores that do not harbour tension-generating attachments. BubR1 is an integral part of MCC and in its absence, SAC control is lost and the SAC protein Mad2 is no longer localized to unattached kinetochores. As a result, aneuploid daughter cells are generated [16] . It was therefore surprising that in mouse oocytes, the knockdown of BubR1 to 25% of endogenous protein levels led to a metaphase I arrest with the SAC protein Mad2 being localized to kinetochores [17] . On the contrary in another BubR1 knockdown study metaphase-to-anaphase transition of meiosis I occurred in an accelerated manner [18] . Furthermore, BubR1 protein was shown to maintain elevated levels of the APC/C activator Cdh1 in prophase I, which is thought to be required for preventing the entry into meiosis I (refs 17 , 18 ). Over expression of BubR1 stabilized Cdh1 and led to the accelerated progression through meiosis I in one [17] , but not the other [18] study. Loss of BubR1 was suggested to result in the loss of Cdh1 in prophase I, and as a consequence increased Cdk1 activity leading to spontaneous entry into meiosis and arrest in metaphase I [17] . The meiotic role of BubR1 seemed therefore at odds with its role in mitosis for generating the MCC and SAC-induced metaphase arrest. In mitosis, BubR1 has an additional, SAC-independent role. Kinetochore-localized BubR1 is required for the stabilization of kinetochore–microtubule interactions by counteracting Aurora B phosphorylation through the recruitment of PP2A (refs 19 , 20 , 21 , 22 , 23 , 24 ). BubR1 may have a similar role in oocyte meiosis I (ref. 17 ), and its loss may prevent the establishment of correct, stable attachments. Indeed, the previous study suggested that kinetochore–microtubule fibres are diminished upon BubR1 knockdown, but it was not addressed whether the same mechanisms as in mitosis are at work in oocytes to stabilize kinetochore fibres [17] . In human oocytes, an important decrease in BubR1 protein levels is observed in oocytes from women closer to menopause, compared with younger women [25] . Decline of BubR1 function in combination with cohesin reduction in older oocytes [3] , [4] , [5] , [6] , [7] may explain the age-dependent elevated error rates in female meiosis. Therefore it is important to understand how BubR1 controls the first meiotic division in mammalian oocytes. In this study we use a conditional knockout approach to analyse oocytes completely devoid of endogenous BubR1 protein. We show here that BubR1 is required for meiotic SAC control, but not prophase I arrest. We find that BubR1 promotes anaphase onset after complete securin degradation and maturation promoting factor (MPF) inactivation. In addition we identify a meiosis-specific role for BubR1 in establishing a stable spindle, which is independent of Aurora B/C and kinetochore localization of BubR1. BubR1 is not required for maintaining GV arrest in oocytes BubR1 H/H mice harbouring only 10% of endogenous BubR1, due to the introduction of an alternative splicing site, have been generated previously [26] . This BubR1 allele in BubR1 H/H mice is flanked by LoxP sequences [26] , which allows the generation of a conditional knockout. To analyse oocytes completely devoid of BubR1 protein we crossed BubR1 H/H mice with a strain expressing the Cre-recombinase from the oocyte-specific Zp3 promoter [27] . Oocytes obtained from BubR1 H/H Zp3-Cre + mice will therefore be called BubR1 Δ/Δ oocytes, and from BubR1 +/+ Zp3-Cre + mice control oocytes. The efficiency of the knockout was checked by reverse transcription quantitative PCR, using three different primer pairs, and mRNA amounts were assessed relative to mRNA coding for the ribosomal protein Rps16. Fully grown oocytes arrested before entry into meiosis I in prophase I (GV or germinal vesicle) stage, and oocytes entering meiosis I (at GVBD or germinal vesicle breakdown) were compared. No marked differences in mRNA levels were detected between GV stage oocytes from different strain backgrounds, or GV and GVBD oocytes. Importantly, no mRNA coding for full length BubR1 was detected in GV or GVBD BubR1 Δ/Δ oocytes ( Fig. 1a ), these oocytes are therefore deleted for BubR1 . Interestingly, we found that wild-type oocytes harbour ∼ 100 times more BubR1 mRNA than mouse embryonic fibroblasts (MEFs) ( Supplementary Fig. 1 ), indicating that transient knockdown approaches may be inherently difficult to target BubR1 in oocytes. 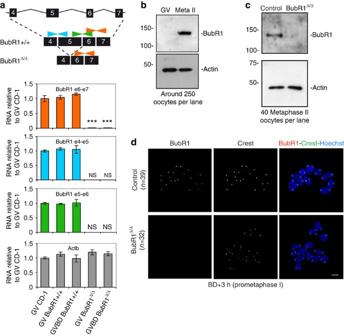Figure 1: No BubR1 mRNA or protein is detected inBubR1Δ/Δoocytes. (a) RNA levels from 20 oocytes were analysed by reverse transcription quantitative PCR normalized to the levels of Rps16 RNA. The position of the three BubR1 primer pairs is indicated in the scheme. Control reactions in which the RT enzyme was omitted were verified to be negative. Graphs show averages normalized to Rps16 and s.e.m. (standard error of the mean) from triplicate samples from a representative experiment. β-Actin was used as an additional internal control. For BubR1 e6-e7 RNA levels, significance of the differences betweenBubR1+/+andBubR1Δ/Δwas estimated using Student’st-test. (mean±s.e.m.; ***P<0.0001; n.s., no signal detected). BubR1 is conditionally deleted inBubR1Δ/Δoocytes. Note: comparable mRNA levels for BubR1 are found in GV oocytes of two different mouse strains, CD-1 and C57Bl6/Sv129. (b) Western blot of GV stage and metaphase II oocytes. The western blot was repeated three times. (c) Western blot of metaphase II (meta II) control andBubR1Δ/Δoocytes. The western blot was repeated two times. (d) Chromosomes spreads of prometaphase I control andBubR1Δ/Δoocytes at GVBD+3 h, stained for BubR1 (red), kinetochores (Crest, green) and chromosomes (Hoechst, blue). The number of oocytes analysed in four independent experiments is indicated. Scale bar, 5 μm. Figure 1: No BubR1 mRNA or protein is detected in BubR1 Δ/Δ oocytes. ( a ) RNA levels from 20 oocytes were analysed by reverse transcription quantitative PCR normalized to the levels of Rps16 RNA. The position of the three BubR1 primer pairs is indicated in the scheme. Control reactions in which the RT enzyme was omitted were verified to be negative. Graphs show averages normalized to Rps16 and s.e.m. (standard error of the mean) from triplicate samples from a representative experiment. β-Actin was used as an additional internal control. For BubR1 e6-e7 RNA levels, significance of the differences between BubR1 +/+ and BubR1 Δ/Δ was estimated using Student’s t -test. (mean±s.e.m. ; *** P <0.0001; n.s., no signal detected). BubR1 is conditionally deleted in BubR1 Δ/Δ oocytes. Note: comparable mRNA levels for BubR1 are found in GV oocytes of two different mouse strains, CD-1 and C57Bl6/Sv129. ( b ) Western blot of GV stage and metaphase II oocytes. The western blot was repeated three times. ( c ) Western blot of metaphase II (meta II) control and BubR1 Δ/Δ oocytes. The western blot was repeated two times. ( d ) Chromosomes spreads of prometaphase I control and BubR1 Δ/Δ oocytes at GVBD+3 h, stained for BubR1 (red), kinetochores (Crest, green) and chromosomes (Hoechst, blue). The number of oocytes analysed in four independent experiments is indicated. Scale bar, 5 μm. Full size image It was previously shown that BubR1 protein accumulates during meiotic maturation [17] , [18] . We compared BubR1 protein levels in oocytes arrested at GV stage with oocytes arrested in metaphase II. Whereas BubR1 was easily detected in metaphase II, protein levels of BubR1 in GV were below detection levels in our hands ( Fig. 1b ). Therefore we used metaphase II oocytes, which contain much more BubR1 protein to ask whether BubR1 protein can still be detected in BubR1 Δ/Δ oocytes. BubR1 was not detected in BubR1 Δ/Δ but in control oocytes by western blot. Because of the difficulties in obtaining a clear BubR1 signal in GV oocytes by immunofluorescence due to the very low protein amounts and diffuse localization, we analysed oocytes in prometaphase I. BubR1 was not detected in BubR1 Δ/Δ oocytes by immunofluorescence in prometaphase I, when endogenous BubR1 starts to accumulate at the kinetochores in control oocytes ( Fig. 1c,d ). We asked whether the loss of BubR1 affected GV arrest and entry into meiosis I (GVBD). BubR1 Δ/Δ oocytes did not enter meiosis I spontaneously in dbcAmp or IBMX-containing medium (both drugs prevent entry into meiosis I), in contrary to BubR1 knockdown oocytes [17] , [18] , nor were efficiencies of entry or timing different from control oocytes ( Fig. 2a–c ). BubR1 Δ/Δ and wild-type oocytes harboured comparable Cdk1 activity before and after entry into meiosis I ( Fig. 2d ), demonstrating that APC/C-dependent degradation of mitotic cyclins, which is thought to maintain GV arrest [28] is not affected in oocytes without BubR1. Therefore we conclude that BubR1 is not required for prophase I arrest in mouse oocytes. 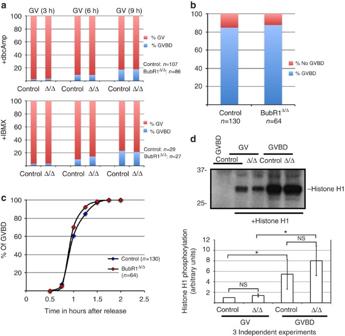Figure 2: BubR1 is not required for GV arrest in mouse oocytes. (a) Percentage of the indicated number of GV control andBubR1Δ/Δoocytes that underwent spontaneous GVBD in the presence of dbcAmp or IBMX in the culture medium, at the indicated times after harvesting, in three independent experiments. (b) Percentage of the indicated number of GV control andBubR1Δ/Δoocytes that did GVBD within 90 min after release, adjusted to 100%, in three independent experiments. (c) Time of GVBD in control andBubR1Δ/Δoocytes after release, in three independent experiments. (d)In vitrokinase assays of control andBubR1Δ/Δoocytes in GV stage and at GVBD, using Histone H1 as a substrate. For quantifications, kinase activity at GV in controls was set to 1 and the mean relative kinase activities of control andBubR1Δ/Δoocytes at GV and GVBD are shown. Error bars indicate±s.d. from three independent experiments, using Student’st-test. (*P<0.05; NS, non-significant). Figure 2: BubR1 is not required for GV arrest in mouse oocytes. ( a ) Percentage of the indicated number of GV control and BubR1 Δ/Δ oocytes that underwent spontaneous GVBD in the presence of dbcAmp or IBMX in the culture medium, at the indicated times after harvesting, in three independent experiments. ( b ) Percentage of the indicated number of GV control and BubR1 Δ/Δ oocytes that did GVBD within 90 min after release, adjusted to 100%, in three independent experiments. ( c ) Time of GVBD in control and BubR1 Δ/Δ oocytes after release, in three independent experiments. ( d ) In vitro kinase assays of control and BubR1 Δ/Δ oocytes in GV stage and at GVBD, using Histone H1 as a substrate. For quantifications, kinase activity at GV in controls was set to 1 and the mean relative kinase activities of control and BubR1 Δ / Δ oocytes at GV and GVBD are shown. Error bars indicate±s.d. from three independent experiments, using Student’s t -test. (* P <0.05; NS, non-significant). Full size image Accelerated progression through meiosis I without BubR1 Next, we wanted to establish whether BubR1 Δ/Δ oocytes progress beyond metaphase I, unlike BubR1 knockdown oocytes [17] . Time-lapse live imaging showed that metaphase I-to-anaphase I transition and polar body (PB) extrusion took place ( Fig. 3a,b , Supplementary movies 1 and 2 ). Similar to what was observed on the loss of other checkpoint proteins such as Mps1 or Bub1 (refs 8 , 12 ), meiosis I was accelerated, chromosomes were not aligned at the metaphase plate ( Fig. 3a–c ) and missegregations occurred in 85% of BubR1 Δ/Δ oocytes, as determined by metaphase II spreads ( Fig. 3d ). In wild-type oocytes, the SAC protein Mad2 is found localized to unattached kinetochores early in prometaphase I (ref. 11 ). Mad2 staining was lost in oocytes without BubR1 ( Fig. 3e ), further showing that the meiotic SAC is defective without BubR1. Indeed, treatment of oocytes with the spindle-depolymerizing drug Nocodazole led to a transient SAC arrest in metaphase I only in oocytes with functional BubR1 ( Fig. 3c ). As expected, exogenously expressed wild-type BubR1, but not the BubR1 E406K (GLEBS) mutant, which cannot interact with Bub3 (refs 29 , 30 ), localized to kinetochores ( Fig. 3f ). Wild-type BubR1 expression rescued Mad2 localization to kinetochores in prometaphase I ( Fig. 3e ), and induced a metaphase I arrest in control and BubR1 Δ/Δ oocytes ( Fig. 3g ), showing that defective SAC control is due to the absence of BubR1. Alignment of chromosomes in BubR1 Δ/Δ oocytes was rescued on the expression of wild-type BubR1, but not by preventing chromosome segregation through the inhibition of APC/C-dependent degradation with the proteasome inhibitor MG132 ( Fig. 3a , Supplementary movies 3-8 ). 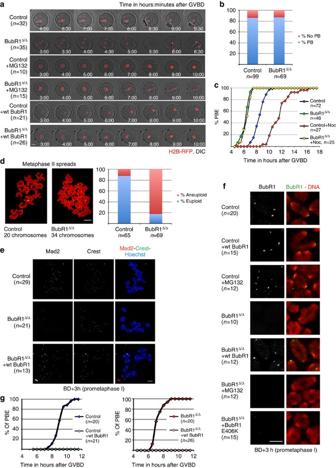Figure 3: Meiosis I is accelerated and SAC control is impaired without BubR1. (a) Selected time frames of representative movies of H2B-RFP injected control andBubR1Δ/Δoocytes undergoing the first meiotic division. Shown are overlays of the stack. Where indicated, mRNA encoding for wild-type (wt) BubR1 was injected at GV stage, or MG132 was added at GVBD+3 h. Scale bar. 20 μm. DIC, differential interference contrast. The indicated number of oocytes has been analysed in at least three independent experiments. (b) Percentage of the indicated number of control andBubR1Δ/Δoocytes extruding PBs, in three independent experiments. (c) Time of PB extrusion in the indicated number of control andBubR1Δ/Δoocytes is adjusted to 100%, in three independent experiments. Nocodazole was added at GVBD+3 h, where indicated. (d) Representative metaphase II chromosome spreads of a control and aBubR1Δ/Δoocyte. Kinetochores were stained with Crest (green), chromosomes with Propidium iodide (red). Scale bar, 5 μm. The number of spreads analysed in three independent experiments is indicated. The graph illustrates that >80% ofBubR1Δ/Δoocytes are aneuploid after the first division. (e) Prometaphase I spreads at GVBD+3 h of control and BubR1Δ/Δoocytes, stained for Mad2 (red), kinetochores (Crest, green) and chromosomes (Hoechst, blue). Scale bar, 5 μm. The number of spreads analysed in three independent experiments is indicated. (f) BubR1 localization (in green) to kinetochores in metaphase I control andBubR1Δ/Δoocytes, after wt BubR1 mRNA injection where indicated. BubR1 E406K was injected intoBubR1Δ/Δoocytes, and kinetochore localization was determined at GVBD +3 h. Oocytes were treated with MG132 at GVBD+3 h where indicated. Kinetochores are visible due to brighter DNA staining. Chromosomes were stained with Hoechst and pseudo-coloured red. Scale bar, 5 μm. The number of spreads analysed in three independent experiments is indicated. (g) Meiotic maturation of control andBubR1Δ/Δoocytes after the injection of wt BubR1 mRNA at GV stage. The number of oocytes analysed in three independent experiments is indicated. Expression of BubR1 prevents PB extrusion. Figure 3: Meiosis I is accelerated and SAC control is impaired without BubR1. ( a ) Selected time frames of representative movies of H2B-RFP injected control and BubR1 Δ/Δ oocytes undergoing the first meiotic division. Shown are overlays of the stack. Where indicated, mRNA encoding for wild-type (wt) BubR1 was injected at GV stage, or MG132 was added at GVBD+3 h. Scale bar. 20 μm. DIC, differential interference contrast. The indicated number of oocytes has been analysed in at least three independent experiments. ( b ) Percentage of the indicated number of control and BubR1 Δ/Δ oocytes extruding PBs, in three independent experiments. ( c ) Time of PB extrusion in the indicated number of control and BubR1 Δ/Δ oocytes is adjusted to 100%, in three independent experiments. Nocodazole was added at GVBD+3 h, where indicated. ( d ) Representative metaphase II chromosome spreads of a control and a BubR1 Δ/Δ oocyte. Kinetochores were stained with Crest (green), chromosomes with Propidium iodide (red). Scale bar, 5 μm. The number of spreads analysed in three independent experiments is indicated. The graph illustrates that >80% of BubR1 Δ/Δ oocytes are aneuploid after the first division. ( e ) Prometaphase I spreads at GVBD+3 h of control and BubR1 Δ / Δ oocytes, stained for Mad2 (red), kinetochores (Crest, green) and chromosomes (Hoechst, blue). Scale bar, 5 μm. The number of spreads analysed in three independent experiments is indicated. ( f ) BubR1 localization (in green) to kinetochores in metaphase I control and BubR1 Δ/Δ oocytes, after wt BubR1 mRNA injection where indicated. BubR1 E406K was injected into BubR1 Δ/Δ oocytes, and kinetochore localization was determined at GVBD +3 h. Oocytes were treated with MG132 at GVBD+3 h where indicated. Kinetochores are visible due to brighter DNA staining. Chromosomes were stained with Hoechst and pseudo-coloured red. Scale bar, 5 μm. The number of spreads analysed in three independent experiments is indicated. ( g ) Meiotic maturation of control and BubR1 Δ/Δ oocytes after the injection of wt BubR1 mRNA at GV stage. The number of oocytes analysed in three independent experiments is indicated. Expression of BubR1 prevents PB extrusion. Full size image A functional SAC is not required for metaphase II arrest Oocytes undergo the first meiotic division, progress into metaphase II and remain arrested in metaphase II (cytostatic factor, (CSF) arrest) until fertilization occurs. The role of SAC proteins in the establishment of CSF arrest was not entirely clear in oocytes and has not yet been addressed with a clean, genetic approach. In Xenopus laevis oocytes, it has been suggested that SAC proteins are required for CSF arrest [31] , [32] , [33] , whereas in mouse oocytes the expression of a dominant negative Bub1 mutant did not perturb CSF arrest [34] . To clarify the SAC’s role in CSF arrest, we asked whether the complete loss of BubR1 affected CSF arrest and release from the arrest. For comparison we additionally analysed CSF arrest in oocytes devoid of functional Mps1 (ref. 12 ), a kinase essential for SAC control in mitosis [14] and meiosis [12] and upstream of other SAC components [14] . Mps1 ΔN/ΔN oocytes harbour only a mutant version of Mps1, which cannot localize to kinetochores but retains its kinase activity. Control, BubR1 Δ/Δ and Mps1 ΔN/ΔN oocytes were induced to undergo meiosis II metaphase-to-anaphase transition with sister chromatid separation. As expected, metaphase II oocytes without functional BubR1 or Mps1 are aneuploid, but otherwise we observed no defect in establishing a CSF arrest or release from the arrest, as judged from the presence of single sisters and no dyads in anaphase II ( Fig. 4 ). Hence we conclude that CSF arrest and release per se do not require SAC proteins. 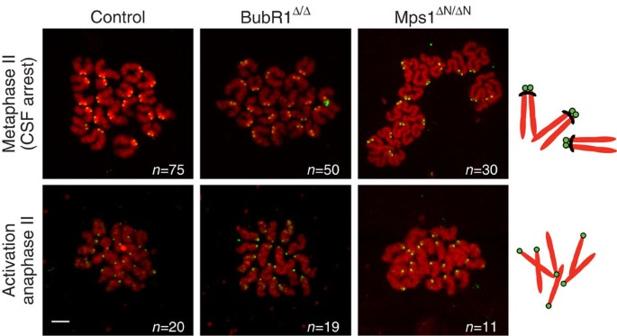Figure 4: Loss of SAC control does not affect metaphase II CSF arrest. Chromosome spreads of control,Mps1ΔN/ΔNandBubR1Δ/Δoocytes in metaphase II (CSF arrest) and anaphase II. Chromosomes were stained with propidium iodide (red), kinetochores with Crest (green). Scale bar, 5 μm. Schemas of the expected chromosome figures for wild-type oocytes are shown on the right. In metaphase II dyads (paired sister chromatids) are held together by centromeric cohesin, which is illustrated in black. Note that only single sister chromatids are present in anaphase II. The number of oocytes analysed in three independent experiments is indicated. Figure 4: Loss of SAC control does not affect metaphase II CSF arrest. Chromosome spreads of control, Mps1 ΔN/ΔN and BubR1 Δ/Δ oocytes in metaphase II (CSF arrest) and anaphase II. Chromosomes were stained with propidium iodide (red), kinetochores with Crest (green). Scale bar, 5 μm. Schemas of the expected chromosome figures for wild-type oocytes are shown on the right. In metaphase II dyads (paired sister chromatids) are held together by centromeric cohesin, which is illustrated in black. Note that only single sister chromatids are present in anaphase II. The number of oocytes analysed in three independent experiments is indicated. Full size image Loss of BubR1 delays anaphase I onset and PB extrusion Interestingly, progression through meiosis I in BubR1 Δ / Δ oocytes was accelerated but not as much as observed on the loss of other checkpoint proteins, such as Bub1 (ref. 8 ) or Mps1 (ref. 12 ). To directly compare meiotic timing in oocytes without BubR1 to oocytes without Mps1 kinase activity we used reversine to inhibit Mps1 kinase activity in the same strain background [35] . Addition of reversine to the culture medium after entry into meiosis led to the same phenotypes we had previously observed in oocytes harbouring only the Mps1ΔN mutant protein [12] . In reversine-treated oocytes, kinetochore localization of Mps1 was not affected as shown by the live imaging of GFP-Mps1 (in accordance with kinase activity of Mps1 being required for its removal from kinetochores [36] ), meiosis I was accelerated as much as in Mps1 ΔN/ΔN harbouring oocytes [12] , Mad2 was absent from kinetochores in prometaphase I, and accordingly, the checkpoint was not functional ( Fig. 5a–c ). 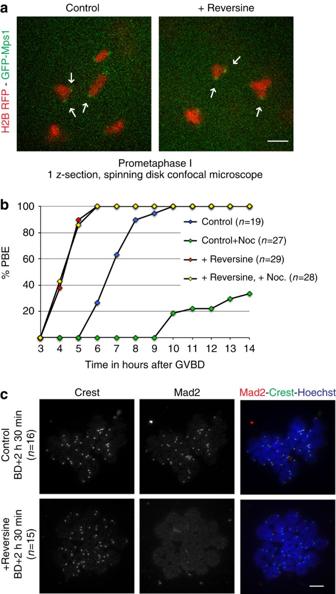Figure 5: Reversine treatment phenocopies loss of kinetochore-localized Mps1. (a) GFP-Mps1 and Histone H2B-RFP (to visualize chromosomes) were expressed in control and reversine-treated oocytes. Reversine was added at GVBD. At GVBD+3 h, GFP-Mps1 localization was analysed by live imaging, using a spinning disk confocal microscope. Only 1 z-section is shown. Scale bar, 5 μm. The arrowheads indicate GFP-Mps1 localized to the kinetochores in this z-section. 10 oocytes in three independent experiments were analysed. (b) Time of PB extrusion in the indicated number of control and reversine-treated oocytes in three independent experiments. Reversine was added at GVBD, Nocodazole was added at GVBD+3 h, where indicated. (c) Prometaphase I spreads at GVBD+2h 30 min of control and reversine-treated oocytes (from GVBD onwards), stained for Mad2 (red), kinetochores (Crest, green) and chromosomes (Hoechst, blue). The number of oocytes analysed in three independent experiments is indicated. Scale bar, 5 μm. Figure 5: Reversine treatment phenocopies loss of kinetochore-localized Mps1. ( a ) GFP-Mps1 and Histone H2B-RFP (to visualize chromosomes) were expressed in control and reversine-treated oocytes. Reversine was added at GVBD. At GVBD+3 h, GFP-Mps1 localization was analysed by live imaging, using a spinning disk confocal microscope. Only 1 z-section is shown. Scale bar, 5 μm. The arrowheads indicate GFP-Mps1 localized to the kinetochores in this z-section. 10 oocytes in three independent experiments were analysed. ( b ) Time of PB extrusion in the indicated number of control and reversine-treated oocytes in three independent experiments. Reversine was added at GVBD, Nocodazole was added at GVBD+3 h, where indicated. ( c ) Prometaphase I spreads at GVBD+2h 30 min of control and reversine-treated oocytes (from GVBD onwards), stained for Mad2 (red), kinetochores (Crest, green) and chromosomes (Hoechst, blue). The number of oocytes analysed in three independent experiments is indicated. Scale bar, 5 μm. Full size image Oocytes without Mps1 kinase activity accelerated meiosis I on average 170 min, whereas oocytes without BubR1 accelerated meiosis I only by 120 min ( Fig. 6a,b ). We asked whether this reflected BubR1-independent SAC activity still present in BubR1 Δ/Δ oocytes, or whether this was indicating an additional role for BubR1 in some other event at the metaphase-to-anaphase transition, independent of the SAC. If the SAC were still active in BubR1 Δ/Δ oocytes, additional inhibition of Mps1 kinase activity with reversine was expected to accelerate PB extrusion, but strikingly, this is not the case ( Fig. 6a,b ). 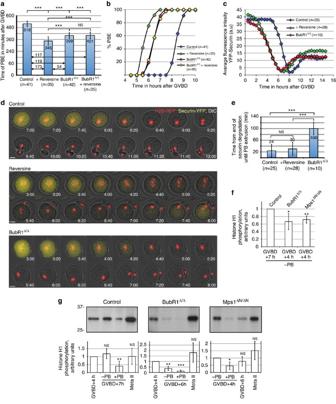Figure 6: Loss of BubR1 delays time from securin degradation and Cdk inactivation until anaphase and PB extrusion. (a) Time of PB extrusion in minutes after GVBD in control, reversine (Mps1 inhibitor)-treated andBubR1Δ/Δoocytes. Where indicated, reversine was added at GVBD. (b) Time of PB extrusion in hours after GVBD in the indicated number of control, reversine-treated,BubR1Δ/Δand reversine-treatedBubR1Δ/Δoocytes, adjusted to 100%. Reversine was added at GVBD. (c) Quantification of YFP-securin signal in control, reversine-treated (from GVBD onwards) andBubR1Δ/Δoocytes during meiotic maturation by live imaging. Representative graphs from three independent experiments are shown and the total number of oocytes analysed is indicated. (d) Selected time frames of representative movies of H2B-RFP and YFP-securin injected control, reversine-treated (from GVBD onwards) andBubR1Δ/Δoocytes undergoing the first meiotic division. 10 z-sections of 3 μm were taken to visualize chromosomes, shown are overlays of the stack. Time points were taken every 20 min, time after GVBD is indicated. (Single channels are shown inSupplementary Fig. 3.). DIC, differential interference contrast. Number of oocytes analysed is shown ine). (e) The time from lowest YFP-securin levels to extrusion of the first PB is indicated in minutes in control, reversine-treated andBubR1Δ/Δoocytes. (f) Quantifications of independentin vitrokinase assays of oocytes 7 h after GVBD (control), or 4 h after GVBD (SAC mutants), using Histone H1 as a substrate. Five control,Mps1ΔN/ΔNandBubR1Δ/Δ, oocytes were used for each time point. See Material and Methods section for quantifications. (g)In vitrokinase assays of control,BubR1Δ/ΔandMps1ΔN/ΔNoocytes at GVBD+ 4 h, before and after PB extrusion, and in metaphase II, using Histone H1 as a substrate. Representative kinase assays are shown for each genetic background, and below are the quantifications of at least three independent experiments each. See Material and Methods section for quantifications. Time after GVBD is indicated in hours. −PB, oocytes that have not yet extruded a PB, +PB, oocytes had just extruded a PB (oocytes were selected individually), Meta II, metaphase II. Error bars ina,e,fandgindicate +/− s.d. from at least three different experiments, using Student’st-test (***P<0.0001; **P<0.001; *P<0.05; NS, non-significant). Figure 6: Loss of BubR1 delays time from securin degradation and Cdk inactivation until anaphase and PB extrusion. ( a ) Time of PB extrusion in minutes after GVBD in control, reversine (Mps1 inhibitor)-treated and BubR1 Δ/Δ oocytes. Where indicated, reversine was added at GVBD. ( b ) Time of PB extrusion in hours after GVBD in the indicated number of control, reversine-treated, BubR1 Δ/Δ and reversine-treated BubR1 Δ/Δ oocytes, adjusted to 100%. Reversine was added at GVBD. ( c ) Quantification of YFP-securin signal in control, reversine-treated (from GVBD onwards) and BubR1 Δ/Δ oocytes during meiotic maturation by live imaging. Representative graphs from three independent experiments are shown and the total number of oocytes analysed is indicated. ( d ) Selected time frames of representative movies of H2B-RFP and YFP-securin injected control, reversine-treated (from GVBD onwards) and BubR1 Δ/Δ oocytes undergoing the first meiotic division. 10 z-sections of 3 μm were taken to visualize chromosomes, shown are overlays of the stack. Time points were taken every 20 min, time after GVBD is indicated. (Single channels are shown in Supplementary Fig. 3 . ). DIC, differential interference contrast. Number of oocytes analysed is shown in e ). ( e ) The time from lowest YFP-securin levels to extrusion of the first PB is indicated in minutes in control, reversine-treated and BubR1 Δ/Δ oocytes. ( f ) Quantifications of independent in vitro kinase assays of oocytes 7 h after GVBD (control), or 4 h after GVBD (SAC mutants), using Histone H1 as a substrate. Five control, Mps1 ΔN/ΔN and BubR1 Δ/Δ , oocytes were used for each time point. See Material and Methods section for quantifications. ( g ) In vitro kinase assays of control, BubR1 Δ/Δ and Mps1 ΔN/ΔN oocytes at GVBD+ 4 h, before and after PB extrusion, and in metaphase II, using Histone H1 as a substrate. Representative kinase assays are shown for each genetic background, and below are the quantifications of at least three independent experiments each. See Material and Methods section for quantifications. Time after GVBD is indicated in hours. −PB, oocytes that have not yet extruded a PB, +PB, oocytes had just extruded a PB (oocytes were selected individually), Meta II, metaphase II. Error bars in a , e , f and g indicate +/− s.d. from at least three different experiments, using Student’s t -test (*** P <0.0001; ** P <0.001; * P <0.05; NS, non-significant). Full size image To get insights into the nature of the supplementary delay observed in BubR1 Δ/Δ oocytes we asked whether the APC/C is activated at the same time in oocytes without Mps1 and BubR1. In other words, we wanted to know whether the delay occurs after checkpoint satisfaction in wild-type oocytes. Inactivation of the SAC leads to APC/C activation and consequently to the accelerated degradation of securin and cyclin B1. YFP-tagged securin can therefore be used as a read-out for APC/C activation and SAC inactivation [8] . Kinetics and timing of yellow fluorescent protein (YFP)-securin degradation in BubR1 Δ/Δ oocytes was indistinguishable from YFP-securin degradation in reversine-treated oocytes, indicating that in both cases the APC/C is not inhibited by the SAC ( Fig. 6c ). Next, we asked whether chromosome segregation was delayed in oocytes without BubR1. Indeed, simultaneous live imaging of YFP-securin degradation and H2B-RFP-labelled chromosomes showed that anaphase I onset and PB extrusion were significantly delayed in oocytes without BubR1, but not in oocytes treated with reversine ( Fig. 6d,e , supplementary Fig. 2 ). Time from anaphase onset till PB extrusion was the same with or without BubR1 ( Fig. 6d , supplementary Fig. 2 ). The delay in BubR1 Δ/Δ oocytes was therefore independent of its role in the SAC, and independent of a potential feedback control for cytokinesis, which has been described recently in mitotic cells [37] . We asked whether Cdk1 is inactivated at the same time in oocytes without either Mps1 or BubR1, and whether throughout the supplementary delay in BubR1 Δ/Δ oocytes Cdk1 activity remains high or low. APC/C-dependent cyclin B1 degradation to reduce Cdk1/cyclin B1 activity is required for metaphase-to-anaphase transition [38] . We performed in vitro kinase assays using Histone H1 as a substrate to determine when Cdk1-cyclin B1 is inactivated. In controls, highest Cdk1 activity in meiosis I was observed at GVBD+7 h, and in both BubR1- and Mps1-deficient oocytes at GVBD+4 h ( Fig. 6f ), even though SAC deficient oocytes never reached the same levels of Cdk1/cyclin B1 activity. Checkpoint-deficient oocytes underwent metaphase-to-anaphase transition with much lower overall Cdk1/cyclin B1 activity ( Fig. 6f ), meaning that in the absence of SAC control less Cdk1/cyclin B1 activity is required for APC/C activation and metaphase-to-anaphase transition. A drop in Cdk1 activity was observed after PB extrusion in control oocytes, and in SAC-devoid oocytes at GVBD+6 h, at which time PB extrusion had occurred in oocytes without functional Mps1, but not in BubR1 Δ/Δ oocytes ( Fig. 6g ). This indicates that endogenous cyclin B has been degraded at the same time in both checkpoint mutants, similar to YFP securin. Importantly, during the supplementary delay observed in BubR1 Δ/Δ oocytes, Cdk1 activity remained low (GVBD+6 h without PB extrusion, Fig. 6g ). We conclude that BubR1 has an additional, SAC-independent role for anaphase I onset. Without BubR1, oocytes delay the separation of chromosomes, even though MPF activity is low and securin has been degraded. Localization of BubR1 to kinetochores in meiosis I Kinetochore localization in mitosis is downstream of Mps1 and Aurora B kinase activities [14] . Mitotic kinetochore localization of BubR1 is required not only for its role in the SAC, but also for stabilizing kinetochore–microtubule attachments, through recruitment of PP2A-B56 which counteracts Aurora B phosphorylation [19] , [23] , [24] . To get insights into the different potential roles of BubR1 in meiosis we asked how kinetochore localization of BubR1 is regulated in oocytes. Endogenous BubR1 was localized to kinetochores in prometaphase I, and weakly in metaphase I when kinetochores are attached ( Fig. 7a,b , the BubR1 signal co-localized with Crest, Fig. 1b ), in agreement with the two previous studies [17] , [18] . BubR1 localization to kinetochores in prometaphase I depends on Mps1 kinase activity, as the signal disappeared in the presence of reversine ( Fig. 7a,b ). Correction of wrongly attached kinetochore–microtubule fibres requires kinetochore recruitment of the Aurora B kinase in mitosis. Aurora B substrate phosphorylation leads to the destablization of kinetochore fibres and to the further recruitment of SAC components to the kinetochore [14] . In meiosis, Aurora B and C are expressed [39] , [40] with Aurora C being mainly responsible for error correction [40] , [41] . Both Aurora B and C can be inhibited with ZM447439 in mouse oocytes [41] . We controlled for the efficiency of the inhibitor by staining for phospho-mitotic centromere-associated kinesin, a known Aurora B substrate ( supplementary Fig. 3a ). BubR1 localization to kinetochores was dependent on Aurora B/C activity in meiosis I ( Fig. 7a,b ). 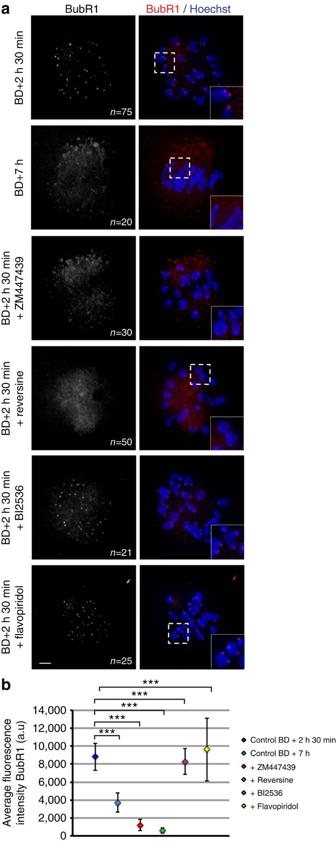Figure 7: Kinetochore localization of BubR1 in meiosis depends on Mps1 and Aurora B/C kinase activities. (a) Whole-mount immunofluorescence staining to detect endogenous BubR1 in wild-type oocytes at GVBD+2 h 30 min (early prometaphase I) or GVBD+7 h (metaphase I). Where indicated, oocytes were treated from GVBD onwards with Mps1 inhibitor (reversine), Aurora B/C inhibitor (ZM447439), Plk1 inhibitor (BI2536) and Cdk inhibitor (flavopiridol), and fixed at GVBD+2 h 30 min. Oocytes were stained with BubR1 antibody (red) and Hoechst (to visualize chromosomes, blue). All stainings were repeated at least three times in independent experiments, and the number of oocytes analysed is indicated. Scale bar, 5 μm. Inserts show magnifications to better see the kinetochore signal. Scale bar, 5 μm. (b) Quantification of BubR1 antibody staining of oocytes ina), as described in Material and Methods. At least 10 oocytes were analysed per condition, from at least three independent experiments. Error bars indicate mean±s.d.; ***P<0.0001, by Student'st-test. Figure 7: Kinetochore localization of BubR1 in meiosis depends on Mps1 and Aurora B/C kinase activities. ( a ) Whole-mount immunofluorescence staining to detect endogenous BubR1 in wild-type oocytes at GVBD+2 h 30 min (early prometaphase I) or GVBD+7 h (metaphase I). Where indicated, oocytes were treated from GVBD onwards with Mps1 inhibitor (reversine), Aurora B/C inhibitor (ZM447439), Plk1 inhibitor (BI2536) and Cdk inhibitor (flavopiridol), and fixed at GVBD+2 h 30 min. Oocytes were stained with BubR1 antibody (red) and Hoechst (to visualize chromosomes, blue). All stainings were repeated at least three times in independent experiments, and the number of oocytes analysed is indicated. Scale bar, 5 μm. Inserts show magnifications to better see the kinetochore signal. Scale bar, 5 μm. ( b ) Quantification of BubR1 antibody staining of oocytes in a ), as described in Material and Methods. At least 10 oocytes were analysed per condition, from at least three independent experiments. Error bars indicate mean±s.d. ; *** P <0.0001, by Student's t -test. Full size image Stabilization of kinetochore–microtubule attachments in mitosis furthermore depends on BubR1 phosphorylation by both Plk1 and Cdk1 kinases [15] . First we controlled for the efficiency of the Plk1 inhibitor BI2536 and the Cdk inhibitor flavopiridol [42] . Interestingly, the addition of the Plk1 inhibitor from GVBD onwards impeded on APC/C activation and PB extrusion, but not checkpoint control ( Supplementary Fig. 3b and c ). (Addition of BI2536 after GVBD+5 h permitted PB extrusion with segregation of sister chromatids in meiosis I, in accordance with a recent study) [43] (data not shown). As expected, treatment with high doses of the Cdk inhibitor flavopiridol [44] inhibited GVBD, as Cdk1 activity is required for entry into meiosis [45] ( supplementary Fig. 3d ). Importantly, though, the treatment with inhibitors against either Plk1 or Cdk1 kinases at these concentrations did not remove BubR1 from kinetochores in meiosis ( Fig. 7a,b ). In summary, we conclude that Aurora B/C and Mps1, but not Plk1 or Cdk1 kinase activities are required for proper kinetochore localization of BubR1 in meiosis I. BubR1 is required for the establishment of stable spindles Now we asked whether BubR1’s role for the establishment of stable kinetochore–microtubule interactions is conserved in meiosis I. Indeed, nearly no cold-stable microtubule fibres attached to kinetochores were detected in oocytes without BubR1 ( Fig. 8a,b ), in agreement with the previous study [17] . On the other hand inhibition of Mps1 with reversine or Aurora B/C with ZM447439 in control oocytes still allowed the establishment of stable kinetochore fibres ( Fig. 8a,b ), even though BubR1 was not localized to the kinetochores ( Fig. 7a,b ). Chromosomes were misaligned in the presence of ZM447439 and upon loss of Mps1 activity, also in agreement with previous literature [12] , [39] , [40] ( Fig. 8a ). Importantly, though, the failure to establish stable kinetochore fibres in BubR1 Δ/Δ oocytes was not rescued by simultaneously inhibiting Mps1, or Aurora B/C, unlike in mitosis [23] . This indicates that the formation of stable kinetochore fibres depends on BubR1, but not on its kinetochore localization to counteract Aurora B/C phosphorylation. It was previously shown that the inhibition of Cdk1 activity during meiosis I leads to a delay, but not the abolishment of stable kinetochore fibres [46] . Treatment of oocytes with Cdk or Plk1 inhibitor still allowed the formation of stable microtubule fibres, showing that unlike in mitosis, BubR1 phosphorylation by Plk1 or Cdk1 is not required for the formation of stable kinetochore fibres ( Fig. 8a,b ). 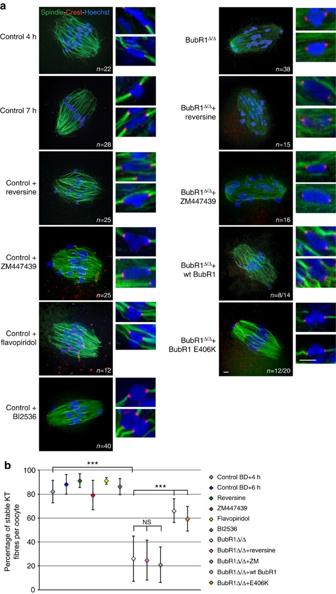Figure 8: Cytosolic BubR1 is required for establishing stable microtubule fibres in meiosis I. (a) Whole-mount immunofluorescence of control oocytes at 4 h and control andBubR1Δ/Δoocytes just before anaphase onset. Where indicated, oocytes were treated with reversine, ZM447439, flavopiridol and BI2536, to inhibit Mps1, Aurora B/C, Cdk1 and Plk1 kinases, respectively, from GVBD onwards, except for ZM447439, which was added 2 h before fixation. For staining of stable microtubule fibres, oocytes were cold-treated on ice for 4–5 min before fixation. One representative oocyte is shown for each condition; the number of oocytes analysed from at least three independent experiments is indicated, as well as the number of oocytes with the phenotype shown. For the rescue, mRNA coding for wild-type (wt) BubR1 or the BubR1 E406K mutant was injected into GV oocytes. To obtain oocytes before anaphase I onset, control oocytes were fixed at GVBD+7 h, except those treated with reversine, which were fixed at GVBD+4 h.BubR1Δ/Δoocytes (with or without reversine or ZM447439) were fixed at GVBD+5 h andBubR1Δ/Δoocytes+wt or E406K BubR1 mRNA at GVBD+6 h. A control at GVBD+4 h is shown as well. Spindles are green (α-tubuline), chromosomes blue (Hoechst), and kinetochores red (Crest serum). Shown are representative overlays of the acquisitions with a spinning disk confocal microscope (20 z-sections every 0,8 μm), from at least three independent experiments. Scale bar. 5 μm. Inserts show zooms of individual z-planes. (b) Quantifications of kinetochores that are attached and shown ina) as described in Material and Methods. At least three independent experiments were analysed for each condition, and the mean percentage of attached kinetochores of at least 12 oocytes was determined by Student’st-test. Error bars show mean±s.d.; ***P<0.0001, NS, non-significant. KT, kinetochore). Figure 8: Cytosolic BubR1 is required for establishing stable microtubule fibres in meiosis I. ( a ) Whole-mount immunofluorescence of control oocytes at 4 h and control and BubR1 Δ/Δ oocytes just before anaphase onset. Where indicated, oocytes were treated with reversine, ZM447439, flavopiridol and BI2536, to inhibit Mps1, Aurora B/C, Cdk1 and Plk1 kinases, respectively, from GVBD onwards, except for ZM447439, which was added 2 h before fixation. For staining of stable microtubule fibres, oocytes were cold-treated on ice for 4–5 min before fixation. One representative oocyte is shown for each condition; the number of oocytes analysed from at least three independent experiments is indicated, as well as the number of oocytes with the phenotype shown. For the rescue, mRNA coding for wild-type (wt) BubR1 or the BubR1 E406K mutant was injected into GV oocytes. To obtain oocytes before anaphase I onset, control oocytes were fixed at GVBD+7 h, except those treated with reversine, which were fixed at GVBD+4 h. BubR1 Δ/Δ oocytes (with or without reversine or ZM447439) were fixed at GVBD+5 h and BubR1 Δ/Δ oocytes+wt or E406K BubR1 mRNA at GVBD+6 h. A control at GVBD+4 h is shown as well. Spindles are green (α-tubuline), chromosomes blue (Hoechst), and kinetochores red (Crest serum). Shown are representative overlays of the acquisitions with a spinning disk confocal microscope (20 z-sections every 0,8 μm), from at least three independent experiments. Scale bar. 5 μm. Inserts show zooms of individual z-planes. ( b ) Quantifications of kinetochores that are attached and shown in a ) as described in Material and Methods. At least three independent experiments were analysed for each condition, and the mean percentage of attached kinetochores of at least 12 oocytes was determined by Student’s t -test. Error bars show mean±s.d. ; *** P <0.0001, NS, non-significant. KT, kinetochore). Full size image Our results pinpoint to the requirement of cytoplasmic BubR1 for the formation of stable microtubule fibres. Therefore we asked whether the establishment of stable fibres in BubR1 Δ/Δ oocytes can be rescued with the BubR1 E406K mutant, which does not localize to the kinetochores ( Fig. 3f ) [29] , [30] . Indeed, stable microtubule fibres are formed in BubR1 Δ/Δ oocytes expressing BubR1 E406K ( Fig. 8 ). Taken together, our data show that BubR1 plays an additional, hitherto unknown direct or indirect role for microtubule stabilization independent of its kinetochore localization, which can be separated from its mitotic role in counteracting Aurora B/C phosphorylation at kinetochores, and which is specific to oocyte meiosis. Women in industrialized countries tend to postpone childbearing, leading to a 70% increase in trisomic pregnancies over 20 years in the United Kingdom [47] . Women in their 40’s have a risk of developing a trisomic pregnancy close to 30%, compared with women in their 20’s with a risk below 5% (ref. 48 ). Trisomy 21 pregnancies (95%) are due to errors in female meiosis [48] , whereas errors in chromosome segregation in male meiosis are much lower, being around 2.5% for autosomes [49] . Unlike meiotic divisions in males, which take place immediately after pachytene and successful recombination, female meiosis comes to a halt for weeks or months (in mice) or decades (in humans) in prophase I, before meiosis is resumed to give rise to one or more fertilizable eggs. Obviously this long arrest poses an important challenge to oocytes and is thought to be one major reason for the high error rate in female meiosis [1] . During this long arrest hardly any cohesin turnover seems to take place, and indeed it has been shown that there is a decrease in the amount of cohesin found on metaphase I chromosomes, which ultimately leads to the weakening of chiasmata and precocious separation of homologues in meiosis I (refs 3 , 5 , 6 , 7 , 50 , 51 ). It has been shown previously that the knockdown of BubR1 in GV oocytes leads to spontaneous [17] or accelerated [18] entry into meiosis I, suggesting a role for BubR1 in GV arrest. The proposed role for BubR1 to maintain the protracted GV arrest was expected to affect fertility because this may lead to precocious depletion of the oocyte stock. Our data here show that, at least in mice, this is not the case and that BubR1 is not required for prophase arrest. Loss of BubR1 also did not affect the number of mature GV oocytes, as was expected if oocytes without BubR1 entered meiosis spontaneously. Instead we find that BubR1 is absolutely essential for generating eggs of the correct ploidy for fertilization. Accordingly, female mice harbouring oocytes devoid of BubR1 are sterile. The loss of BubR1 accelerates meiosis because of the loss of SAC control, but it slows down the time from complete securin degradation and MPF inactivation to anaphase onset and PB extrusion. Spindles in oocytes without BubR1 do not contain detectable stable microtubule fibres, and we show here that cytosolic BubR1 plays a role in stabilizing microtubule fibres. This function of BubR1 is independent of its known mitotic role in counteracting Aurora B and independent of Plk1 or Cdk1 phosphorylation of BubR1. We do not yet know why BubR1 Δ/Δ oocytes delay anaphase I onset, but it is attractive to speculate that unstable fibres physically prevent anaphase movements and PB extrusion. In mitotic cells, BubR1-associated PP2A-B56 was shown to promote chromosome movements to the metaphase plate and the formation of stable kinetochore fibres by counteracting HSET/kinesin-14, a minus end directed motor protein [52] . It remains to be addressed whether in meiosis BubR1-associated PP2A targets this and other motor proteins, in a kinetochore-independent manner. We do not think that the supplementary delay of BubR1 Δ/Δ oocytes for anaphase I onset is due to a failure to dephosphorylate Knl1 that has been previously phosphorylated by Mps1 (ref. 53 ), because reversine treatment did not revert the observed delay. Alternatively, PP2A-B56 associated with BubR1 may be important to counteract other phosphorylation events in the cytoplasm or at the spindle that prevent anaphase onset, and in the absence of BubR1, anaphase I onset takes more time because of delayed dephosphorylation of certain substrates that remain to be identified. How can we explain the discrepancies of our study with the two previous studies on BubR1’s role for maintaining GV arrest [17] , [18] ? Apart from potential off-target effects that can occur with any RNA interference approach, the knockdown efficiencies can be highly variable between individual oocytes and depend on the amount of morpholino-oligo injected in each oocyte and on the incubation times. Neither study has examined on a single-cell level the variability of the knockdown. Furthermore, our data show that levels of mRNA coding for BubR1 are quite high in oocytes of the two different mouse strains that we compared, relative to MEFs (see also NCBI, UniGene, EST Profile Viewer, for Bub1b) and relative to mRNA levels of actin or Rps16, making a transient knockdown approach extremely difficult. Therefore, we think that the discrepancies for BubR1’s role in GV arrest are due to technical reasons related to the knockdown approach. The differences between our study and the previous transient knockdown studies on BubR1’s role for progression through meiosis I and localizing Mad2 to kinetochores, are also most likely due to the incomplete knockdown of BubR1. The partial depletion of BubR1 may affect the stability of the spindle, but not abolish checkpoint control, in which case oocytes will fail to correctly attach kinetochores and activate the SAC, leading to the observed metaphase arrest with Mad2 at kinetochores described by Homer et al . [17] . On the other hand, Wei et al . [18] reported an accelerated progression through meiosis I, in line with our results. The variability of the phenotypes observed is most likely due to different knockdown efficiencies in the two studies. A functional SAC should recognize a failure to establish tension-bearing attachments that is due to age-related decline of cohesin, in meiosis, but there are several reasons why this may not be the case (ref. 1 ): (1) a single univalent may biorient at the meiotic spindle and evade the checkpoint because tension-bearing attachments can be established such as in mitosis, (2) a mono-oriented univalent attached to one pole is not recognized because the meiotic SAC may not sense whether attachments are also under tension from both the poles, (3) the spindle checkpoint is not as sensitive as in mitosis, and a single unattached or not correctly attached kinetochore may not be recognized, (4) activation of the SAC leads only to a transient arrest in metaphase, and ultimately oocytes will exit checkpoint arrest and missegregate chromosomes and (5) the SAC may become weaker with age. Indeed, reduced transcription of the SAC proteins BubR1, Bub1 and Mad2 and reduced protein levels of BubR1 have been observed in aged human oocytes [25] , [54] . Whether the SAC is indeed—at least in part—responsible for the observed age-related increase in chromosome missegregations in aged oocytes is a subject of controversy. One previous study was using a senescence accelerated mouse strain, with a premature decline in fertility. Oocytes of these artificially aged mice have troubles aligning their chromosomes at the metaphase plate and meiosis I is accelerated, indicating that the SAC is not fully functional [55] . On the contrary in another study, oocytes of naturally aged oocytes had a functional checkpoint and did not show an acceleration of anaphase onset, indicating that increased missegregations with age are not due to a missing spindle checkpoint [56] . Functionality of the checkpoint was examined by treating oocytes with low doses of Nocodazole, and one can argue that even a weakened checkpoint may still respond to Nocodazole, but not recognize a few unattached kinetochores in metaphase I. Oocytes from CBA/Ca mice that also show a premature decline in fertility, missegregate chromosomes at high rates but do not accelerate meiosis I, either [51] . Importantly, a recent study using standard C57Bl6/J laboratory mice and comparing young with naturally aged mice showed reduced rates of the SAC protein Mad2 at the kinetochores of oocytes from older mice, weakened checkpoint response upon Nocodazole treatment, increased incidence of misaligned chromosomes, but normal timing of meiosis I (ref. 57 ). The normal timing of meiosis I in these mice and CBA/Ca mice is therefore not necessarily the best indicator for checkpoint functionality: more chromosome misalignments in oocytes of older mice may lead to a weak checkpoint response, which will get overridden, but make it impossible to detect a potential acceleration of meiosis I (ref. 57 ). A conclusion from these studies is that functionality of the SAC with age is differently affected in different mouse strains, and not all mouse strains are equally suited to study the involvement of the SAC in the increase of missegregation events in oocytes of older mice [57] . Overall these results suggest that the SAC is functional in oocytes of older mice and still able to generate a delay in anaphase I onset, but that it becomes less efficient with age and this leads to an increase in chromosome missegregations. To get better insights into how the age-related drop in BubR1 protein levels may affect chromosome segregation in mammalian oocytes it was necessary to analyse oocytes completely devoid of BubR1. This allowed us to distinguish the roles of BubR1 for SAC control, the formation of stable spindle fibres and anaphase onset. SAC control seems to be more permissive in meiosis than mitosis, and therefore less BubR1 in older oocytes will affect chromosome segregation, not only because of its role in the checkpoint, but also because of its checkpoint-independent functions in meiosis. In the light of our study, the observed age-related decline of BubR1 in human oocytes [25] in combination with a gradual loss of cohesin [3] , [4] , [5] , [6] , [7] is expected to have severe consequences on chromosome segregation and therefore fertility in humans. Mouse strains, husbandry and genotyping Mice were maintained and bred in the animal facility of UMR7622 according to local rules by the French Ministery of Higher Education and Research, and ethical approbation, in compliance with the application of the rule of the ‘3 Rs’ (License 5330). The number of mice used was kept as low as possible but high enough to obtain statistically significant results, in agreement with the standards used in the field. Prophase I oocytes were harvested from 9–11-week-old mice as described below. BubR1 H/+ mice [26] on a mixed C57Bl6/Sv129 background were crossed with Z p3-Cre (C57BL/6-Tg(Zp3-Cre)93Knw/J) mice (The Jackson Laboratories; USA). For every experiment, oocytes from BubR1 H/H Zp3-Cre + mice ( BubR1 Δ/Δ oocytes) were compared with the corresponding oocytes from BubR1 +/+ Zp3-Cre + littermates (control oocytes). For replicate experiments mice from different litters were used. Genotyping was performed as published [26] using the following primers: BubR1-1 (forward): 5′- GTA AGT CTA TTT CTC CTG GAT TAA GTA G -3′, BubR1-2 (reverse): 5′- CAT CTG TGT ACC ATA CGT GTG TCT GG -3′, BubR1-3 (reverse): 5′- ATA TTG CTG AAG AGC TTG GCG GCG -3′. Cre presence was determined according to the protocol provided by The Jackson Laboratories. Mps1ΔN/ΔN mice have been characterized previously [12] . CD-1 (Swiss) mice (Janvier, France) were used for experiments not involving BubR1 H/H Zp3-Cre + mice. Reverse transcription semi-quantitative PCR Reverse transcription and real time semi-quantitative PCR were carried out as described in ref. 12 , from 20 oocytes or 500 ng of RNA from MEF cells, with the following modifications: qPCR reactions were performed in 20 μl using the Brilliant III ultra fast SYBR Green Kit (Agilent Technologies). Primer sequences for BubR1 are: BubR1-e5F: 5′- AGGAAGGGATTGAACGCAAG -3′; BubR1-e6R: 5′- ATTCCCAAGGGCCAAGAAAG -3′; BubR1-e4F: 5′- CAAGGAGAGACGCGCTATTAT -3′; BubR1-e5R: 5′- TAGAACTGGGCAAGGGAAAC -3′; BubR1-e6F: 5′- GAAGAGCAGAGGGAAGAAGATG -3′; BubR1-e7R: 5′- AAACGGTGATCCTGCGATTA -3′. Primer sequences for β-actin are: Actb-F: 5′- CATTGCTGACAGGATGCAGAAGG -3′; Actb-R: 5′- TGCTGGAAGGTGGACAGTGAGG -3′. Primer sequences for Rps16 are published in ref. 12 . Oocyte culture and drug treatments Oocytes were harvested from ovaries of sexually mature female mice and cultured in self-made M2 medium droplets containing dibutyryl cyclic AMP (dbcAMP, Sigma; 200 μM), unless otherwise described. Follicle cells were removed by carefully mouth-pipetting oocytes through a torn-out pasteur-pipette with a diameter allowing easy entry of individual oocytes. Only oocytes entering meiosis I within 90 min after release were used for the experiments. Oocyte activation in metaphase II was done by incubating metaphase II oocytes in CaCl 2 -free M2 medium supplemented with 10 mM SrCl 2 (ref. 58 ). Different drugs for this study were used at the following concentrations: IBMX (3-isobutyl-1-methylxanthine, Sigma-Aldrich): 100 μM; Nocodazole (Sigma-Aldrich): 0.3 μM; Reversine (Merck Chemicals Ltd.): 0.5 μM; ZM447439 (Santa Cruz): 20 μM; BI2536 (Selleckchem): 0.2 μM; Flavopiridol (Sigma-Aldrich): 1 μM, MG132 (Sigma-Aldrich): 20 μM. Drugs were added to the culture medium and for all drugs, the time of addition and duration of treatment are indicated. Because oocytes are cultured in drops covered with mineral oil and because reversine is soluble in oil, mineral oil covering the culture drops contained reversine as well, and untreated controls were cultured in separate dishes. Chromosome spreads, whole-mount immunofluorescence Antibody staining of chromosome spreads and fixed oocytes [58] , [59] , was done using the following antibodies at the indicated dilutions: BubR1 polyclonal sheep antibody (gift from S. Taylor, 1/50), human CREST auto-immune antibody (Cellon SA, HCT-0100; 1/100), mouse monoclonal α-tubulin (DMA1) coupled to FITC (Sigma-Aldrich, F2168; 1/100), rabbit polyclonal MCAK-phospho S95 (Abcam, ab74146;1/50) and Mad2 polyclonal rabbit antibody [60] , 1/100). The following secondary antibodies were used: CY3 anti rabbit (Jackson ImmunoResearch, 711-166-152; 1/200), CY3 anti sheep (Jackson ImmunoResearch, 713-165-147; 1/200) and anti human Alexa 488 (Life Technologies, A11013; 1/200). Cold-stable spindles were obtained by incubating oocytes on top of an ice-water bath for 5 min before fixation [58] . Acquisitions of antibody staining on fixed oocytes were done with an Olympus IX70 Spinning Disk Confocal microscope (100x/1.2 NA objective, triple pass filter set, Sutter excitation filter wheel, MicroMax cooled CCD (charge-coupled device) camera (Princeton Inst.) and Metamorph software [58] . In vitro transcription, microinjections and live imaging In vitro transcription of YFP securin, Histone H2B-RFP, GFP-Mps1 (ref. 12 ), BubR1 E406K (ref. 61 ) and wild-type mouse BubR1 (ref. 61 ) were performed with the Ambion mMessage Machine kit and 1–10 pM of mRNAs purified on RNAeasy columns (Qiagen) were microinjected with Eppendorf micromanipulators on a Nikon Eclipse Ti microscope and a FemtoJet microinjector [58] . The murine BubR1 E406K plasmid was a kind gift of L. Malureanu (Mayo Clinic, MN, USA). For live imaging, a motorized inverted Nikon TE2000E microscope (Plan APO 20 x/0.75 NA objective) was used, equipped with PrecisExite High Power LED Fluorescence (LAM 1: 400/465, LAM 2: 585), a temperature chamber (Life Imaging Services), a Märzhäuser Scanning Stage, a CoolSNAP HQ2 camera, and controlled by Metamorph software. Live imaging of GFP-Mps1 was done on an Olympus IX70 Spinning Disk Confocal microscope as above (100x/1.2 NA objective; ref. 12 ). Oocytes were cultured in Ludin chambers (Life Imaging Services) [12] , [58] . Western blots, kinase assays Western blots were performed using the indicated number of oocytes at specific stages [58] . For western blot detection the following antibodies were used: Actin (ab3280, 1/200) and BubR1 (Sheep polyclonal antibody, S. Taylor, 1/200). For the BubR1 western blots using 250 oocytes per lane (corresponding to oocytes from ∼ 8 mice) we re-used membranes previously used to detect Cyclin A with a different antibody [58] , to comply with the rule of the 3R’s for animal research, using the same internal control (actin). HeLa cells used as controls were treated with 12 ng ml −1 Nocodazole for 18 h and extracts were prepared in NP40 buffer [62] . Super Signal West Femto Maximal Sensitivity Substrate (Thermo Scientific) and recommended secondary antibodies were used. Whole membranes for Fig. 1b,c are shown in Supplementary Fig. 1b and c . Kinase assays to check overall MPF activity were done on aliquots of five oocytes at the indicated stages of meiotic maturation, using Histone H1 (Sigma) as a substrate [11] . In short, oocytes were lysed in 3 μl NP-40 lysis buffer [62] , and kinase reactions were performed in 6 μl final volume for 30 min at 30 °C (ref. 11 ). Incorporation of radioactivity was detected by SDS–PAGE (as an example a different exposure of the whole gel of the kinase assay in Fig. 1d is shown in Supplementary Fig. 1d ), and quantitated using Image J software. Quantifications and statistical analysis Fluorescence intensity of signals at kinetochores ( Fig. 7 ) were calculated the following way: first, 5 × 5 pixel circles were manually placed over the kinetochore and the summed pixel values of a given channel calculated. Another 5 × 5 circle was placed adjacent to this to calculate background signal, which was then subtracted from the kinetochore signal. Twenty-five to forty centromeres were calculate per cell using mean grey value measurement in Image J. Samples of sufficient size were used. For any given experiment, at least 10 oocytes were analysed per condition, from at least three independent experiments, using mice from different litters, and statistical significance was determined with Student’s t -test. In each histogram, values are given as mean±s.d. For quantification of kinetochore–microtubule attachments ( Fig. 8 ), for each kinetochore visible due to positive staining with Crest serum the attachment status was determined by analysing the individual z-sections. For each oocyte the ratio of attached versus unattached kinetochores was calculated. At least three independent experiments were analysed for each condition, and the mean percentage of attached kinetochores of at least 12 oocytes was determined. Statistical significance was determined with Student’s t -test, error bars indicate mean ±s.d. Quantifications of YFP-securin degradation ( Fig. 6 ) were done in Image J from original acquisitions of one constant focal plane. The background substracted [12] . For quantifications of kinase assays in Fig. 2d , values were normalized to control at GV, in Fig. 6f ; to the control at GVBD+7 h; and in Fig. 6g to the wild-type control at GVBD+ 4 h, which were set to 1. For each reaction, five oocytes were pooled and used for each individual time point. Statistical analysis was performed by Student’s t -test. (NS, non-significant, * P <0.05, ** P <0.001, *** P <0.0001). Error bars indicate mean±s.d. How to cite this article: Touati, S. A. et al . Mouse oocytes depend on BubR1 for proper chromosome segregation but not prophase I arrest. Nat. Commun. 6:6946 doi: 10.1038/ncomms7946 (2015).